Atomic Auger Doppler effects upon emission of fast photoelectrons Studies of photoemission processes induced by hard X-rays including production of energetic electrons have become feasible due to recent substantial improvement of instrumentation. Novel dynamical phenomena have become possible to investigate in this new regime. Here we show a significant change in Auger emission following 1 s photoionization of neon, which we attribute to the recoil of the Ne ion induced by the emission of a fast photoelectron. Because of the preferential motion of the ionized Ne atoms along two opposite directions, an Auger Doppler shift is revealed, which manifests itself as a gradual broadening and doubling of the Auger spectral features. This Auger Doppler effect should be a general phenomenon in high-energy photoemission of both isolated atoms and molecules, which will have to be taken into account in studies of other recoil effects such as vibrational or rotational recoil in molecules, and may also have consequences in measurements in solids. It is a standard assumption that as a first approximation the kinetic energy of electrons emitted during Auger decay depends on the energy difference between the electronic levels involved in the relaxation process, but does not correlate with the photon energy inducing the primary photoionization process. Furthermore, the Auger peak shape and fine structure are also assumed in general to be independent of the primary photon energy. However, there are some effects that can cause detectable changes in the Auger kinetic energy and/or peak shape in specific photon energy ranges. The most well-known example is the post-collision interaction (PCI) effect, which enhances the Auger electron kinetic energy and causes asymmetry of the Auger peak shape when the photon energy is only slightly above the ionization threshold. As the photon energy further increases, the Auger peak reaches the asymptotic energy and gains a symmetric shape (see for example refs 1 , 2 , 3 , 4 , 5 ). In rare cases, there are some specific photon energies where an overlap with other structures of different origin (see for example ref. 6 ), or the interaction with continuum resonances modifying the vibrational distribution of the photoelectron line (see for example ref. 7 ) can be observed. Finally, in molecules with inversion symmetry Cohen-Fano oscillations cause photon-energy-dependent Auger spectra [8] . In the photoionization process, the outgoing electron carries a momentum that is identical but opposite to the momentum of the remaining atom, molecule or solid. However, because of energy and momentum conservation, in molecules and solids the recoil energy can also be stored in the vibrational or rotational degrees of freedom, or in the recoil of the entire solid. For molecules, such recoil effects have been described for the first time in the pioneering work by Domcke and Cederbaum [9] . They are, however, rather weak in the soft X-ray regime up to about 1 keV in energy and have been observed only in recent years in photoelectron spectra: the first observation of vibrational recoil was observed by Kukk et al. [10] in the methane molecule. Later on, this effect was more clearly observed in the tetrafluoro methane molecule CF 4 (ref. 11 ). Another manifestation of vibrational recoil was observed in Ne dimers, and it was shown that a significant modification of the nuclear dynamics accompanying interatomic Coulomb decay is induced by the recoil momentum imparted on the nuclei by fast photo- and Auger electrons [12] . Some years later rotational recoil was also observed [13] . Using hard X-rays of several keV in energy, the recoil effect was also observed in the valence [14] and core ionization [15] of solids. Another reported observation of Doppler phenomenon in electron emission is the rotational Doppler effect, where the rotational motion of an object affects the energy of emitted radiation. Rotational Doppler broadening has been theoretically predicted [16] and observed in high-resolution photoelectron spectroscopy [17] . We here demonstrate that Doppler effects in high-energy photoemission at energies well away from any resonances can significantly affect Auger emission. In particular, we report a phenomenon showing a marked variation in Auger lineshape, depending on the direction with respect to the detector, which we interpret as a manifestation of the Doppler effect due to ion recoil after emission of an energetic photoelectron. Experimentally observed Ne Auger lines The heart of our observations is an unprecedented change in Auger emission following 1 s photoionization of neon, which we attribute to the recoil of the ion induced by the emission of an energetic photoelectron. More in detail, when the photoelectron is emitted from the Ne 1 s shell, with high enough kinetic energy, the recoil ‘kick’ imparted to the ion pushes it mainly in two opposite directions because the differential photoelectric cross-section of the 1 s photoelectron results via dipole selection rules in a p-wave that is oriented along the electric-field vector ( E vector of the incoming radiation, assuming linear polarization). Thus, the photoelectron is emitted preferentially along these two p-lobes, 180 degrees apart. Another way of saying this is that the dipole asymmetry parameter is 2 (ref. 18 ). The Auger electrons that are emitted following the 1 s ionization therefore take off from recoiling ions that are statistically moving in opposite directions. In our system, the Auger electrons are collected from ions travelling towards the detector or away from it. This is the origin of a Doppler shift that we observe as a gradual broadening and doubling of the Auger spectral features. A pictorial representation of the phenomenon is shown in Fig. 1 . 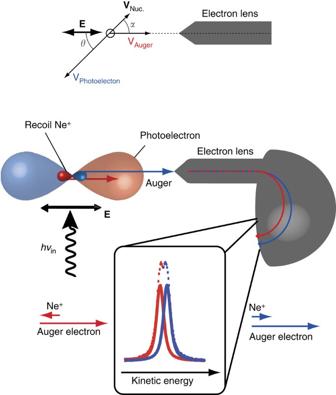Figure 1: Schematic diagram of the physical phenomenon and of the experimental set-up. The polarization vectorEof the incoming synchrotron radiation light is along the detection axis. The lengths of the velocity vectorsvdo not indicate realistic ratios of the velocities. Figure 1: Schematic diagram of the physical phenomenon and of the experimental set-up. The polarization vector E of the incoming synchrotron radiation light is along the detection axis. The lengths of the velocity vectors v do not indicate realistic ratios of the velocities. Full size image The observed splitting into two components is similar to that predicted by Gavrilyuk et al. [19] theoretically for fluorescence spectra. In the present case, the Ne Auger final state after the photoionization of a 1 s electron is reached by the emission of two 2 p electrons. The remaining doubly charged neon ion possesses a total spin of zero and an angular momentum of two; in atomic physics, this situation is also described with a so-called 1 D 2 symmetry. The experimentally observed photon-energy dependence of the Ne 1 s −1 →2 p −2 ( 1 D 2 ) line is simulated with a simple model providing a very good agreement with the experiment, see Methods. In addition, we show that this effect opens the opportunity to measure for photon energies in the keV regime the electron angular distribution including non-dipole effects. 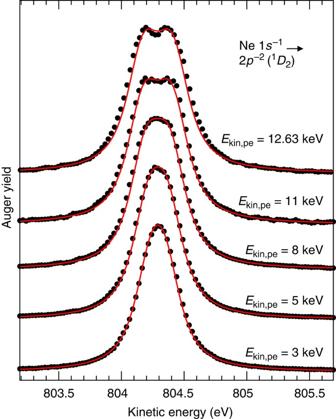Figure 2: The Ne 1s−1→2p−2(1D2) Auger transition. The spectra show the results measured subsequent to photoionization with different kinetic energies of the photoelectron between 3 keV and 12.63 keV. The solid line through the data points is a simulation based on a simple model described in the text. Figure 2 shows the Ne 1 s −1 →2 p −2 ( 1 D 2 ) Auger transition at a kinetic energy of 804.30 eV (ref. 20 ) measured following Ne 1 s −1 photoionization with kinetic energies of the photoelectron between 3 keV and 12.63 keV. We have selected this Auger transition only because the corresponding peak is intense and well separated, but our observations hold for the entire Auger spectrum. Clearly, the lineshape broadens with increasing kinetic energy of the photoelectron, finally resulting in a double peak at high energies. None of the previously mentioned explanations for a photon energy dependence in Auger spectra explains our results, since we are very far above the photoionization threshold and no continuum or discrete resonances play a role. Instead, we propose a mechanism based on the kinematics of the photoelectron and subsequent Auger decay. The essence of the phenomenon is the following: the incoming photons ionize the Ne 1 s electrons (ionization potential 870.17 eV (ref. 21 )). The photoelectrons are ejected in two cones around the E vectors showing the p-wave cos 2 angular distribution, since the initial state is a 1 s orbital with β =2. The ions left behind recoil in two opposite directions and must show a velocity that, because of momentum conservation, depends on the kinetic energy of the ejected photoelectrons (see Fig. 1 ). Our detection system is fixed at a position with the main axis parallel to the E vector and collects Auger electrons emitted from ions travelling towards or away from the detector resulting in blue- and red-shifted kinetic energies, respectively. The energy difference between the red- and blue-shifted components depends on the ion recoil, since the Auger kinetic energy is constant in the atomic frame. The recoil energy increases with the photon energy and leads to the broadening and eventual splitting of the Auger spectral line. This effect is simulated by a simple model; its result is indicated with the red solid lines in Fig. 2 . Figure 2: The Ne 1 s −1 →2 p −2 ( 1 D 2 ) Auger transition. The spectra show the results measured subsequent to photoionization with different kinetic energies of the photoelectron between 3 keV and 12.63 keV. The solid line through the data points is a simulation based on a simple model described in the text. Full size image The simulations are performed with β =2 due to the 1 s ionization and describe an inhomogeneous broadening effect. Because of this, the results have to be convoluted with a Lorentzian of 250 meV (FWHM) for the lifetime broadening of the Ne 1 s level [22] . To simulate the exact lineshape of the Auger transition, the result has to be convoluted with a Gaussian of 100 meV (FWHM) to take into account the present experimental resolution. The good agreement of the simulation with the experimental results demonstrates the quality of the presented model. The Doppler effect in electron emission has been previously observed in the special case of ultrafast fragmentation following core excitation in isolated molecules [23] , [24] , [25] . However, the origin of such Doppler splitting is different from the present case, since it originates from the kinetic energy released by ultrafast dissociation. In more detail, a strongly dissociative potential energy curve of a light molecule may lead to dissociation before the Auger decay and to high kinetic energies of the atomic fragments. If the geometry of the experiments allows selecting one particular direction of fragmentation, then the velocity of these core-excited fragments is either added to or subtracted from the velocity of the emitted resonant Auger electron, resulting in splitting of the Auger lines [23] , [24] , [25] . Such an observation is therefore restricted to ultrafast dissociation of molecules and is not related to the effect we have seen. The Doppler splitting we observe in the Auger electron emission is simply the effect of the velocity of the emitted photoelectrons, if such velocity can be rendered high enough. Our observation is general and not limited to a particular aspect of photoemission dynamics. Simulated Ne and Ar Auger lineshapes One application of this atomic Auger Doppler effect is the determination of unknown angular distributions for high-energy photoelectrons. Because of the difficulty to detect such electrons, these angular distributions are rarely measured at energies high above threshold (see for example, Ne 2 p up to 1,200 eV above threshold [26] ). At these high energies, non-dipole effects are expected to occur. One has to distinguish between first-order non-dipole effects that cause a forward/backward asymmetry in the angular distribution [27] , [28] and second-order non-dipole effects that influence also the plane perpendicular to the propagation direction of the light [18] ; note that this plane is traditionally referred to as the dipole plane. We first discuss the influence of the second-order non-dipole effects, since they are expected to contribute in the present detection plane. The results for the simulation of the Ne 1 s −1 →2 p −2 ( 1 D 2 ) Auger decay subsequent to photoionization with 50.87 keV photons for both, a detection direction parallel (0°) and perpendicular (90°) to the polarization direction are presented in Fig. 3a . The black lines show simulations based on the dipole approximation with β =2 and the red lines by taking the second-order non-dipole effects into account; for details of the non-dipole simulations and for the definition of the second-order non-dipole parameters Δ β , λ , μ and ν relevant in this context, see Equations 6 and 7 in Methods. The latter simulations are based on a linear extrapolation of the second-order non-dipole parameters calculated by Derevianko et al. [18] and show in the 0° spectrum a clear influence. 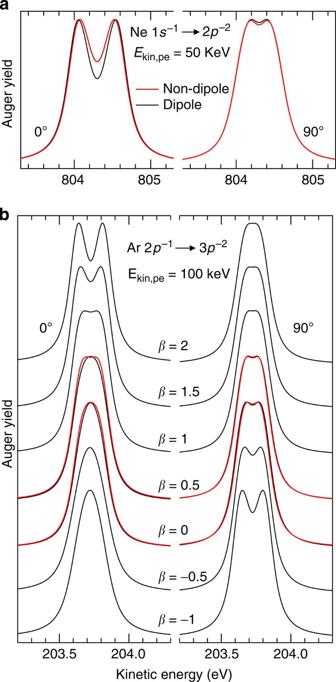Figure 3: Simulations of Auger lineshapes as a function of angular distribution parameters. (a) The Ne 1s−1→2p−2(1D2) Auger transition at a kinetic energy of 50 keV and (b) the Ar 2p−1→3p−2Auger transition at a kinetic energy of 100 keV for the photoelectron. For argon the lineshapes are simulated as a function of theβparameter. The black lines indicate simulations within the dipole approximation while the red lines take second-order non-dipole effects into account; for more details, see text. The simulations are performed for a detection direction parallel (0°) and perpendicular (90°) to the polarization direction of the synchrotron radiation. Figure 3: Simulations of Auger lineshapes as a function of angular distribution parameters. ( a ) The Ne 1 s −1 →2 p −2 ( 1 D 2 ) Auger transition at a kinetic energy of 50 keV and ( b ) the Ar 2 p −1 →3 p −2 Auger transition at a kinetic energy of 100 keV for the photoelectron. For argon the lineshapes are simulated as a function of the β parameter. The black lines indicate simulations within the dipole approximation while the red lines take second-order non-dipole effects into account; for more details, see text. The simulations are performed for a detection direction parallel (0°) and perpendicular (90°) to the polarization direction of the synchrotron radiation. Full size image As a second example, we simulated the Ar 2 p −1 →3 p −2 Auger transitions subsequent to a photoionization with 100 keV photons. In this case not only the second-order non-dipole parameters Δ β , λ , μ and ν but also the dipole parameter β is unknown. Therefore, we simulated in a first step in the dipole approximation the lineshapes as a function of β ; the results are displayed by the black lines in Fig. 3b . For the simulations, a lifetime broadening of 115 meV (FWHM) [22] and an experimental resolution of 50 meV (FWHM) was assumed. In a second step, the simulations were performed by using a linear extrapolation of the second-order non-dipole parameters calculated in ref. 18 , see red lines in Fig. 3b . Note that for these simulations β stands for β +Δ β , since one cannot distinguish experimentally between these two quantities. Furthermore, the simulations are limited to β +Δ β =0.5 and 0, since the requirement that P ( θ , φ ) has to be positive leads for the second-order non-dipole parameters to the restrictions −1+ μ + λ ≤ β +Δ β ≤2+ λ −2 μ . The results show in the 0° and in the 90° spectra an opposing trend in their dependence on β as well as an influence of the second-order non-dipole contributions on the lineshapes in the 0° spectra. By taking into account the equality λ + μ + ν =0 (ref. 18 ) all presented lineshapes can be described with only three angular distribution parameters, namely β +Δ β , λ and μ . As a consequence, the suggested method opens the possibility to study the angular distribution in the second-order non-dipole approximation. The great advantage of this method is that it is much easier experimentally to determine the angular distribution by measuring relatively slow Auger electrons instead of a direct measurement of very fast photoelectrons of 50 or 100 keV. As discussed above, the first-order non-dipole effects lead to a forward/backward asymmetry in the ionization process. The asymmetry should be experimentally accessible by a detection direction parallel to the propagation direction of the synchrotron radiation that leads in equation 4 to an additional term proportional to cos α . The resulting asymmetric peaks should permit obtaining information on the non-dipole parameters γ and δ (ref. 29 ). Another application of the Doppler effect in atomic Auger spectra is the measurement of the hard X-ray radiation polarization, assuming the angular distribution parameters are known. There is now-a-days an important development of radiation sources using a laser plasma accelerator in the few hundreds keV energy range [30] . In this energy range, the Doppler splitting in the Auger spectra can become very high (for example, 2 eV for the Ne 1 s −1 →2 p −2 ( 1 D 2 ) Auger transition at 500 keV) and the structures are separated, allowing the polarization to be determined, again, as in the previous example, by measuring relatively slow Auger electrons instead of very fast photoelectrons. In summary, we have observed and simulated the influence of the translational recoil effect on the lineshape of the Ne 1 s −1 →2 p −2 ( 1 D 2 ) Auger transition. This Auger Doppler effect should be a general phenomenon in high-energy photoionization of atoms, molecules and solids, and has to be taken into account in studies of other recoil effects like vibrational or rotational recoil in molecules photoionized with high photon energies. We also have pointed out that this effect has potential applications such as measuring high-energy photoelectron angular distribution parameters or the polarization direction of light sources, both in the high photon energy regime. Experimental set-up The results were obtained at the SOLEIL Synchrotron, France on the GALAXIES beamline, with the newly operational endstation dedicated to hard X-ray photoelectron spectroscopy [31] . Linearly polarized light is provided by a U20 undulator and monochromatized by a Si(111) double crystal. Electrons are analysed by a large acceptance angle EW4000 Scienta hemispherical analyser, whose lens axis is set collinear to the X-ray polarization in fixed geometry. Model for the Auger lineshape The model derives the distribution of the Doppler shift based on the recoil effect, the angular distribution of the photoelectron, and the geometry of the experimental set-up, and shall now be described. With v nuc and v e being the velocity of the nucleus and the electron, respectively, the Doppler shift Δ E Dop observed in the electron spectrum is given by On the right hand side is neglected due to υ nuc ≪ υ e . To specify the Doppler shift for Auger spectra, Δ E Dop,Aug , we first have to derive the velocity v nuc based on the momentum of the emitted photoelectron, p pe . The latter quantity is given in the relativistic regime by with E kin,pe being the kinetic energy of the photoelectron. This results in Here e pe describes the unit vector in the direction of the velocity of the photoelectron, m e and m nuc are the masses of the electron and the nucleus, respectively, and E kin,eff = E kin,pe (1+ E kin,pe /2 m e c 2 ) is an effective kinetic energy that takes relativistic effects into account; note that the last term allows estimating the relativistic corrections by giving E kin,pe in eV and the mass in eV c −2 , that is, 2 m e c 2 =1,022 keV. In a similar way, however, without relativistic corrections, the velocity of the Auger electron amounts to . In the following, we shall specify the Doppler shift observed in the Auger spectra. Here m nuc = M nuc ·1,836· m e , with M nuc being the atomic mass number, and α is the angle between the trajectory of the emitted Auger electron and the nucleus (see Fig. 1 ). Equation 3 can readily be solved for the angle α . In the next step, we will derive a formula for the probability that a given angle α occurs. This magnitude depends on the probability of a given velocity v nuc =− v pe . The probability of the velocities pointing into a solid angle d Ω=sin θ d θ d φ is given by with θ being the angle between the polarization direction of the synchrotron radiation and the emission direction of the photoelectron (see Fig. 1 ). Moreover, σ 0 is the total cross-section. To rewrite P ( θ , φ ) as a function of P ( α ) the relationship between α and θ , φ has to be established. As can be seen in Fig. 1 , the angle α is identical to the angle between the detection direction d and v nuc . In a coordinate system using the polarization direction of the synchrotron light as the z-axis and the propagation direction of the light as x-axis: In the present case, the detection direction is parallel to the polarization direction and we obtain cos α = d · v nuc /| v nuc |=cos θ , that is, α = θ . By replacing θ in Equation 4 with the expression for α derived from Equation 3 one obtains the probability of a given Doppler shift, P (Δ E Dop,Auger ). In case of a detection direction perpendicular to the polarization and the propagation direction axis of the incoming radiation, one obtains cos α =sin θ sin φ , that is, θ =asin((cos α )/(sin φ )) is a function of α and φ . Using this expression in equation 4 and following the procedure described for parallel detection leads again to P (Δ E Dop,Auger ). The influence of the non-dipole parameters In the second order non-dipole approximation with P 2 (cos θ ) and P 4 (cos θ ) being the second order and fourth order Legendre polynomial, respectively. Here, γ , δ , Δ β , λ , μ and ν are the non-dipole parameters for the angular distribution defined in ref. 18 . The first order non-dipole parameters γ and δ cancel out in case of a detection in the dipole plane. The detection parallel to the polarization direction of the light is most suited to show this, since in this case one can simply integrate over φ and obtain By using this expression for P ( θ ) in Equation 4 the remaining second order non-dipole effects can readily be taken into account in the simulations. How to cite this article: Simon, M. et al. Atomic Auger Doppler effects upon emission of fast photoelectrons. Nat. Commun. 5:4069 doi: 10.1038/ncomms5069 (2014).